Hydrogen-free graphene edges Graphene edges and their functionalization influence the electronic and magnetic properties of graphene nanoribbons. Theoretical calculations predict saturating graphene edges with hydrogen lower its energy and form a more stable structure. Despite the importance, experimental investigations of whether graphene edges are always hydrogen-terminated are limited. Here we study graphene edges produced by sputtering in vacuum and direct measurements of the C–C bond lengths at the edge show ~86% contraction relative to the bulk. Density functional theory reveals the contraction is attributed to the formation of a triple bond and the absence of hydrogen functionalization. Time-dependent images reveal temporary attachment of a single atom to the arm-chair C–C bond in a triangular configuration, causing expansion of the bond length, which then returns back to the contracted value once the extra atom moves on and the arm-chair edge is returned. Our results provide confirmation that non-functionalized graphene edges can exist in vacuum. The functionalization and structural engineering of edges are reported to greatly influence the properties of mesoscopic graphene structures [1] , [2] , [3] , [4] , [5] , [6] , [7] . A variety of elements are known to attach to the edge of graphene, such as N, O, H, Fe and Si. However, to date hydrogen has been the most elusive to study due to its small atomic mass. The attachment of hydrogen to graphene edges and its influence on the properties of graphene has been extensively studied theoretically [1] , [8] , [9] , [10] , [11] , [12] , [13] , [14] . Experimentally, the localized energy states at the edges of graphene have been probed at the atomic level by scanning tunnelling microscopy (STM) combined with scanning tunnelling spectroscopy (STS), as well as scanning transmission electron microscopy (STEM) combined with electron energy loss spectroscopy (EELS). STM and STS with sub-nanometre resolution have revealed the dependence of electronic structure on local edge atom configurations [15] , [16] , [17] , [18] , [19] , [20] . STEM with EELS from single carbon edge atoms in graphene showed the existence of unique energy states not found in the bulk [21] . Several energy states were resolved and associated with different edge terminations such as Klein, zig-zag and arm-chair edges. However, it is not possible to obtain an EELS signal from a single H atom at the edge of graphene. Furthermore, when the EELS is acquired at the edge of graphene, the atomic structure may have changed from the initial STEM image used to determine the EELS acquisition region and this makes exact correlations between edge atomic structure and EEL spectra challenging. The edges studied by Suenaga and Koshino [21] were created by electron beam irradiation under vacuum in the TEM and a similar approach to creating edges in graphene has been used in several other reports [22] , [23] , [24] , but the issue of whether hydrogen is attached to the edge atoms has not been probed experimentally. The attachment of hydrogen to either zig-zag or arm-chair edges of graphene changes the local charge density within bonds and should lead to modifications of the C–C bond lengths of the edge atoms relative to non-hydrogen attachment. Kawai and Koga [25] in their theoretical study suggested H-free arm-chair edges reconstruct and form a triple bond on the arm-rest position. This reconstruction gives a predicted bond length reduction from 1.38 to 1.23 Å, which is close to the triple bond of acetylene (1.20 Å). Therefore, by accurately measuring the position of carbon atoms and subsequently determining the C–C bond length in arm-chair graphene edges it should be possible to indirectly determine whether they are hydrogenated. Despite the progress made in scanning probe microscopy (STM and atomic force microscopy) and aberration-corrected transmission electron microscopy (AC-TEM) [26] , [27] , [28] , [29] , [30] , detecting bond length changes at the edges of graphene has been extremely difficult due to the need to fully resolve individual carbon atoms. Recent advances in monochromation of the electron source have enabled AC-TEM with ~80 pm spatial resolution at the low accelerating voltage of 80 kV (refs 26 , 31 ). We recently demonstrated how this leads to the ability to fully resolve individual atoms in graphene, permitting the precise measurement of C–C bond changes within 5–7-membered ring dislocations and monovacancies [32] , [33] . The irradiation of graphene with an electron beam with an energy of 80 keV is known to cause the opening of holes through chemical etching from surface impurities [34] . Once a hole has been opened in graphene the edge atoms are susceptible to further sputtering because the 80 keV energy electrons have sufficient energy to knock out the edge atoms. This results in the subsequent expansion of these holes by sputtering of edge atoms. Carbon atoms at the edge of graphene can also be mobile, and move rapidly between positions of fixed stability leading to edge reconstruction. The rate of edge sputtering is dependent upon the beam current density (BCD), and here we reduced the BCD sufficiently such that the rate of hole expansion was very slow, ~1.4 pm s −1 , and therefore the atomic configuration of the edge structures were stable enough to be sequentially imaged multiple times and an average image formed with high signal to noise contrast from individual atoms. This has enabled the observation of several different types of edge terminations such as zig-zag, Klein edge, arm-chair and reconstructed 5–7 edge structures. In this report, we utilize sub-Angstrom imaging of graphene edges by monochromated AC-TEM at an accelerating voltage of 80 kV, combined with density functional theory (DFT) calculations to examine arm-chair edge structures that are predicted to have shortened C–C bond lengths when they are not functionalized by hydrogen or other atoms [12] , [25] . Time-dependent images capturing a single atom attaching to the arm-chair graphene edge are obtained and reveal real-time changes in bond length due to functionalization. 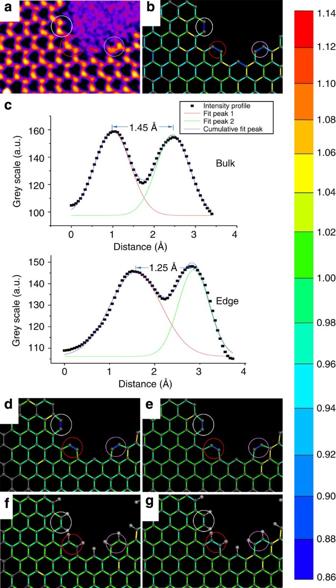Figure 1: Arm-chair edge bond length mapping. (a) AC-TEM image from averaging three consecutive frames with identical structure. The scale bar on the right expresses the amount of compression or elongation of a C–C bond by different colours, the blue end of the spectrum is compression and the red end elongation. The amount of compression or elongation is expressed as a ratio (R) determined by measuring each individual bond length (Bi) and dividing it by a non-perturbed pristine C–C bond length value (Bc–c). See supporting information for further details. This results in contracted bonds have a ratio <1, elongated bonds have a ratio >1 and non-perturbed bonds have ratio ~1. (b) Measured bond lengths expressed in ratio value (R) and represented using the colour scale, from the AC-TEM image in (a). (c) Measurement of bond lengths at the edge (red circled bond inFig. 1a) and in the bulk of graphene by fitting the boxed line profile from two atoms forming a C–C bond with two Gaussians. (d) Colour representation of measured bond length ratios from multi-slice simulated image (including residual aberrations discussed inSupplementary Figs 1–4) based on the DFT calculated atomic structure shown in (e). (e) Colour representation of bond length ratios calculated using DFT. (g) Colour representation of measured bond length ratios from DFT calculations of a hydrogen-terminated structure. (f) Colour representation of measured bond length ratios from a multi-slice simulated image based on the DFT calculated atomic structure shown in (g) (including residual aberrations discussed inSupplementary Figs 1–4). Arm-chair edge bond length mapping Figure 1a is a TEM image of a hole being sputtered on a pristine sheet of graphene by 80-kV electron beam irradiation. This image was formed by averaging three successive frames where the position of atoms had not deviated. This indicates that this specific edge configuration was stable under electron beam irradiation for at least 30 s. Figure 1b shows the measured bond lengths obtained from analysis of the TEM image in Fig. 1a , presented as a ratio that is calculated by dividing each measured bond length by a standard C–C bond length value measured in a non-perturbed region of graphene. Colour scale representation is used in Fig. 1b to display the bond length ratios on the atomic models for ease of visual inspection. The bond lengths were determined by fitting boxed line profiles of two atoms forming the bond with two Gaussians, shown in Fig. 1c , whereby the peaks of the Gaussians were used as the centre of the atomic positions. Contraction of the bond lengths is observed for the three arm-chair bonds at the graphene edge, indicated with blue colour. The ratio between these three bonds and the average bond lengths from the bulk lattice in our images are within the range 0.86–0.88, matching the theoretical predictions found in Kawai and Koga [25] for hydrogen-free arm-chair edges of graphene. We conducted geometrical optimization using DFT for an atomic structure based on the TEM image in Fig. 1a . Bond lengths were measured on both the DFT atomic model shown in Fig. 1e and from the multi-slice simulated image shown in Fig. 1d . Both images show the same shortening of the C–C bond distance, which match the results from the TEM image in Fig. 1a . This confirms that the significant shortening of the C–C bond at the arm-chair edge is due to bond reconstruction rather than an artifact of the TEM imaging. Figure 1: Arm-chair edge bond length mapping. ( a ) AC-TEM image from averaging three consecutive frames with identical structure. The scale bar on the right expresses the amount of compression or elongation of a C–C bond by different colours, the blue end of the spectrum is compression and the red end elongation. The amount of compression or elongation is expressed as a ratio ( R ) determined by measuring each individual bond length ( B i ) and dividing it by a non-perturbed pristine C–C bond length value ( B c–c ). See supporting information for further details. This results in contracted bonds have a ratio <1, elongated bonds have a ratio >1 and non-perturbed bonds have ratio ~1. ( b ) Measured bond lengths expressed in ratio value ( R ) and represented using the colour scale, from the AC-TEM image in ( a ). ( c ) Measurement of bond lengths at the edge (red circled bond in Fig. 1a ) and in the bulk of graphene by fitting the boxed line profile from two atoms forming a C–C bond with two Gaussians. ( d ) Colour representation of measured bond length ratios from multi-slice simulated image (including residual aberrations discussed in Supplementary Figs 1–4 ) based on the DFT calculated atomic structure shown in ( e ). ( e ) Colour representation of bond length ratios calculated using DFT. ( g ) Colour representation of measured bond length ratios from DFT calculations of a hydrogen-terminated structure. ( f ) Colour representation of measured bond length ratios from a multi-slice simulated image based on the DFT calculated atomic structure shown in ( g ) (including residual aberrations discussed in Supplementary Figs 1–4 ). Full size image Prior theoretical work suggests that graphene edges should be very easily passivated with hydrogen as this lowers the edge energy [12] . For comparison, another set of DFT studies were performed, but this time with the graphene edges terminated by hydrogen atoms. Analysis techniques similar to those used in Fig. 1d,e for the hydrogen-free case were applied to the hydrogenated case. Figure 1f shows the measurements of bond lengths from the multi-slice TEM image simulation based on the DFT model and Fig. 1g presents the bond lengths determined from the DFT-calculated atomic structure. The most significant changes occur for the bonds circled with different colours in Fig. 1b,d–g . The arm-chair edge bonds for the hydrogen attached to the edge of graphene, circled in Fig. 1f,g , show no apparent shortening, with one bond even showing a slight elongation in panel (f). Overall, our experimental data from AC-TEM shown in Fig. 1a,b match the case of hydrogen-free edge terminations and we can rule out the presence of hydrogen within these bonds. The s.d. for the TEM bond length ratio measurement was 0.03 Å. This was obtained by measuring >20 C–C bond length values in pristine regions of graphene that was unperturbed and calculating the mean and then the s.d. of the data set relative to the mean value. It is therefore not abnormal to see the slight colour variation in the bulk of the lattice. The bond length ratio of the arm-rest position on the arm-chair edge relative to pristine graphene is on the level of 0.86–0.90, which is well above the noise level. The s.d. values for the DFT model are 0.002 Å and 0.004 Å for hydrogen-free and hydrogen-terminated structures, respectively. These values are calculated in a similar way to the TEM bond ratios, but reflect the uncertainty in the DFT calculation. They are diminutive and thus there is much less colour variation in Fig. 1e,f . The s.d. values for the multi-slice image simulations based on the DFT models are 0.015 Å and 0.013 Å, respectively, for Fig. 1e,g primarily due to the experimental uncertainty introduced Fig. 1d,f in the measurement of the atom positions by line profile analysis. In order to ensure our measurements in Fig. 1 were valid, we repeated the same analysis on a second newly created edge structure, shown in Fig. 2 . The TEM image in Fig. 2a is the average from three images, and Fig. 2b shows the Gaussian fits to line profiles. In Fig. 2c , the bonds of interest are circled and, as in Fig. 1 , they too show shortening. This further confirms that the outermost bonds for the arm-chair edge structure in sputtered graphene edges show C–C bond compression of ~0.86–0.9, which agrees with the predicted bond lengths for triple bonded C≡C and indicates they are free from hydrogen attachment. 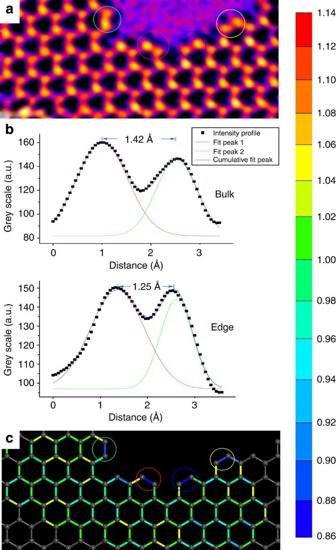Figure 2: Bond length mapping of a second graphene edge. (a) Averaged AC-TEM image from three consecutive frames having identical structures. The scale bars on the right hand side have identical meaning as inFig. 1. (b) Measurement of bond lengths for bulk C–C pairs and for a pair of atoms at the edge in arm-chair configuration using two Gaussian fits to a boxed line profile. (c) Colour representation of bond length ratios for the experimental AC-TEM image in (a). Figure 2: Bond length mapping of a second graphene edge. ( a ) Averaged AC-TEM image from three consecutive frames having identical structures. The scale bars on the right hand side have identical meaning as in Fig. 1 . ( b ) Measurement of bond lengths for bulk C–C pairs and for a pair of atoms at the edge in arm-chair configuration using two Gaussian fits to a boxed line profile. ( c ) Colour representation of bond length ratios for the experimental AC-TEM image in ( a ). Full size image Functionalization-induced bond length changes Tight-binding molecular dynamic (TBMD) simulations revealed that a transient single carbon atom can temporarily functionalize the arm-chair graphene edge to form a unique a triangular edge state, shown in the calculations in Fig. 3 . Functionalization of the arm-chair edge should perturb the C≡C bond and therefore modify the bond length. 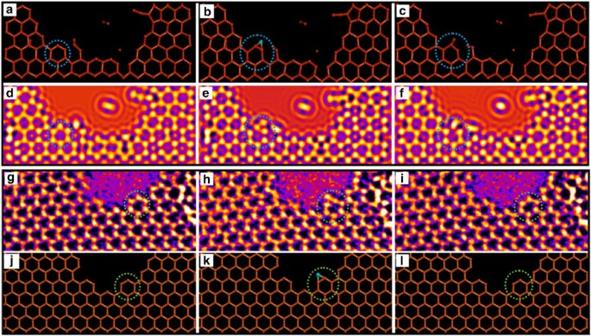Figure 3: Time-dependent functionalization of graphene edges. (a) and (c) are the frames found from molecular dynamic simulation that were prior and after the occurrence of the triangle edge structure that could be seen in (b). (d–f) are multi-slice image simulations based on the atomic models in (a–c) respectively. (g–i) are three consecutive TEM images (20 s between each image) showing the occurrence of the triangle edge structure. (j–l) are atomic models based on the respective TEM images above. Figure 3a–c shows three frames from the TBMD simulation, as atomic models, that reveal the triangular edge state formation, along with corresponding multi-slice image simulations in Fig. 3d–f . The blue dotted circles show the region where the triangle structure appears in Fig. 3b . The blue-coloured atom within the circle is used to identify the extra atom compared with the previous frame. Figure 3c shows the deconstruction of the triangle structure by breaking one of the bonds connecting to the hexagon, and its transformation into a Klein edge on the arm-chair configuration. These TBMD simulations were conducted without the presence of hydrogen, and Fig. 3b shows that the seven atoms within the blue circle prefer to adopt a hexagon–triangle structure instead of opening up to form a heptagon structure under these hydrogen-deprived conditions. Multi-slice image simulations utilizing different microscope conditions reveal that the triangular edge structure can only be resolved with near sub-Angstrom spatial resolution (see Supplementary Fig. 5 ), which is achievable with our monochromated AC-TEM system. While observing the electron beam-induced sputtering of holes in graphene we have recorded the unique triangular edge structure predicted from the TBMD simulation. Figure 3g–i shows a time-series of TEM images with ~20 s between frames, depicting the emergence of the triangular edge structure, with the respective models below them. The triangular structure observed in Fig. 3h is rare and only lasted one frame (~2 s) before being lost. However, since the triangle structure must exist for an appreciable portion of the image exposure time of 2 s it must at least be meta-stable and occupy a local minimum in edge energy. Figure 3: Time-dependent functionalization of graphene edges. ( a ) and ( c ) are the frames found from molecular dynamic simulation that were prior and after the occurrence of the triangle edge structure that could be seen in ( b ). ( d – f ) are multi-slice image simulations based on the atomic models in ( a – c ) respectively. ( g – i ) are three consecutive TEM images (20 s between each image) showing the occurrence of the triangle edge structure. ( j – l ) are atomic models based on the respective TEM images above. 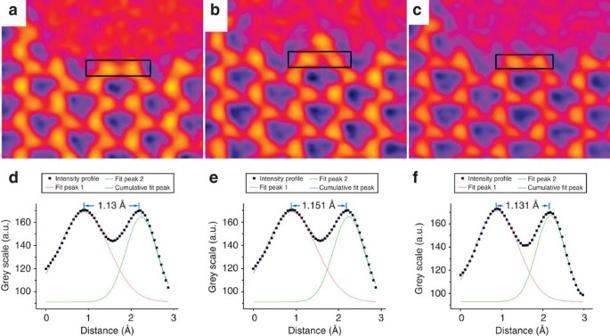Figure 4: Triangle structure analysis. (a–c) Smoothed and false coloured AC-TEM image sequence on the occurrence of the triangle structure (20 s between images, 2 s acquisition time). (d–f) Boxed line profiles from the regions marked in (a–c) with fitted Gaussian profiles for bond length measurements. The bond lengths of the frames before, on and after the occurrence of triangle are marked above the curves. Full size image Figure 4 shows the time-series of AC-TEM images from Fig. 3g–i in greater detail along with their bond length measurements. The triangle–hexagon structure could be interpreted as an arm-chair edge structure being functionalized with an extra atom. Figure 4a–c shows three frames for (a) before, (b) functionalized and (c) after the attachment of the single atom. Box line profiles were taken from the black rectangle area marked in Fig. 4a–c , and are shown in Fig. 4d–f . The three measured bond lengths reveal a change with the addition of an extra atom. The bond length increased from its contracted value of 1.31 Å ( Fig. 4a,d ) to an expanded value of 1.51 Å when the edge is functionalized with a single atom ( Fig. 4b,e ), then returns back to its original contracted length when the extra atom has detached ( Fig. 4c,f ). These results confirm that we are able to detect variations in the distance between the same two carbon atoms in real-time and demonstrate that local bonding variations at the edge are disturbed by atomic functionalization. Figure 4: Triangle structure analysis. ( a – c ) Smoothed and false coloured AC-TEM image sequence on the occurrence of the triangle structure (20 s between images, 2 s acquisition time). ( d – f ) Boxed line profiles from the regions marked in ( a – c ) with fitted Gaussian profiles for bond length measurements. The bond lengths of the frames before, on and after the occurrence of triangle are marked above the curves. Full size image TEM can reveal the location of atoms with the lattice structure of graphene, which in turn can be used to determine the distance between atoms and the C–C bond lengths in graphene. Bond lengths in graphene are dependent upon the electronic charge density within the C–C bonds and therefore large changes in the charge density within graphene C–C bonds can lead to changes in the position of atoms that can be detected using AC-TEM with high spatial resolution. We use this property to show that hydrogen is not attached to the outermost bond of the arm-chair edge, indicating the formation of a triple bond, rather than the saturation of free edge states by hydrogen passivation. This was further confirmed by real-time tracking of the bond lengths, where elongation occurred from functionalization by an additional atom to form a triangular edge state, followed by the contraction of the same C–C bond when the additional carbon was removed. These observations provide strong evidence that the edges of graphene are not always hydrogenated, which is important information for the design of future graphene electronic devices. Synthesis and transfer of graphene The graphene samples were grown by chemical vapour deposition using a liquid copper catalyst as previously reported [35] . This was achieved by placing a high-purity copper sheet (Alfa Aesar, Puratonic 99.999% pure, 0.1 mm thick, ~1 cm 2 ) on top of a similar sized piece of molybdenum (Alfa Aesar, 99.95% pure, 0.1 mm thick). This was loaded into the quartz tube of the split-tube furnace chemical vapour deposition system, which was subsequently sealed, pumped to vacuum and filled with argon. The gas flow was set to 100 s.c.c.m. H 2 /Ar (20% gas mix) and 200 s.c.c.m. pure Ar, and the furnace was ramped to 1090 °C, whereupon the sample was slid into the hot zone of the furnace. The sample was annealed for 30 min, after which the CH 4 flow (1% gas mix in Ar) was set to 10 s.c.c.m. and the H 2 /Ar flow reduced from 100 to 80 s.c.c.m., while maintaining the pure argon gas line flow at 200 s.c.c.m. The conditions were maintained for 90 min to obtain continuous film growth. After this, CH 4 flow was disabled and the sample immediately removed from the furnace hot zone, allowing for rapid cooling in the H 2 and Ar atmosphere. A (8% wt. in anisole, 495 molecular weight) PMMA was spin coated onto the graphene side of the sample at 4,700 r.p.m. for 60 s, and then cured at 180 °C for 90 s. The underlying molybdenum and copper were etched away by floating the sample on iron (III) chloride+hydrochloric acid solution for 3 days, until just a transparent PMMA/graphene film remained suspended on the surface. This was then cleaned by floating onto fresh DI water and 30% hydrochloric acid respectively and then cleaned in DI water again. The film was then transferred to a holey silicon nitride TEM grid (Agar Scientific Y5385). Once left to dry for about 3 hours, the sample was baked on a hot plate for 15 min to remove water and improve sample adhesion with the wafer. The sample was then placed in a furnace at 350 °C overnight to remove the PMMA scaffold. Transmission electron microscopy and image processing HRTEM was performed using Oxford’s JEOL JEM-2200MCO field-emission gun TEM, using a CEOS imaging aberration corrector and an accelerating voltage of 80 kV. A double Wien filter monochromator with a 5-μm slit was used to reduce the energy spread of the electron beam to ~0.21 eV. Data were recorded using a Gatan Ultrascan 4 K × 4 K CCD camera with 1–2 s acquisition times. Supplementary Fig. 6 shows (a) the phase plate due to residual aberrations and (b) the tableau of 21 diffractograms taken with different incident beam tilts taken before image acquisition. The following details the residual aberrations of the JEOL 2200MCO HRTEM. Defocus: (C1)=−204±2 nm, twofold astigmatism: (A1)=2±2 nm, threefold astigmatism: (A2)=23±16 nm, coma: (B2)=26±15 nm, 3rd order spherical aberration: (C3)=−1.162±07 μm, fourfold astigmatism: (A3)=278±170 nm, star aberration: (S3)=267±70 nm, fivefold astigmatism: (A4)=32±3 μm. It must be noted that these values are acquired at a magnification of × 500,000 and drift in real time, therefore they may not represent the exact values when the microscope is at a magnification of × 2,000,000, when images of graphene are obtained. Supplementary Fig. 1a–f demonstrates the impact different astigmatism amplitudes have on the resultant image; the values range from 0 to 1.0 nm with an interval of 0.2 nm. Based on the study, twofold astigmatism eventually degrades the resolution of the image and care must be taken to minimize its impact through continual correction. It also possesses a unidirectional stretching effect on graphene lattice. Comparison of Supplementary Fig. 1 with the AC-TEM image shown in Fig. 1a enables an estimated value of 0.2 nm to be obtained. A study on the direction of the astigmatism was carried out, shown in supplementary Fig. 1g–o to accurately define full-detailed profile of the astigmatism; a direction value of 225° was estimated for Fig. 1a . Supplementary Fig. 2 presents multi-slice image simulations of graphene lattice for different values of threefold astigmatism, but with the twofold astigmatism set at 0.2 nm and a direction of 225°, as previously estimated from Supplementary Fig. 1 . After analysis of these images and comparison to Figs 1 and 2 in the main text we estimate the amplitude and direction of the threefold astigmatism to be 40 nm and 315° for the AC-TEM images in Figs 1 and 2 . Supplementary Fig. 3 shows multi-slice image simulations with different values of axial coma, including twofold astigmatism of 0.2 nm and 3-fold astigmatism of 40 nm. A value of 60 nm and 315° was estimated for the axial coma amplitude and directions. Having carefully examined the three major first- and second-order aberrations individually, we combined all aberrations into one simulation ( Supplementary Fig. 4 ) to demonstrate the overall effect on the images of graphene. Supplementary Fig. 4a shows the TEM image of Fig. 1 in the main text and Supplementary Fig. 4b shows the multi-slice image simulation of the representative atomic structure with all aberration values set to 0. Supplementary Fig. 4c shows the new multi-slice image simulation that contains aberration values (twofold=0.2 nm at angle 225°, threefold=40 nm at angle 315° and axial coma=60 nm at angle 315°) estimated by comparing Fig. 1 in the main text with the set of simulations performed in Supplementary Figs 1–3 . The simulation result, based on a DFT relaxed geometry combined with appropriate residual aberrations, was then used to calculate bond lengths across the image as in Fig. 1 . Supplementary Fig. 5 shows the multi-slice image simulations of a DFT relaxed atomistic model, under different defocus spread values while keeping other parameters constant. The defocus spread value changes from 3 to 5, 7 and 9 nm progressively. The value of 3 nm is equal to the microscope setting when the monochromator is turned and a value of 9 nm is similar to normal aberration-corrected conditions. The values of 5 nm and 7 nm represent the evolution of the image simulation regards to the change of defocus spread. Under a value of 3 nm setting, as can be seen from Supplementary Fig. 5b,f , all the atoms could be fully resolved including the extra atom on top of the hexagon that makes up the triangle structure. Under the value of 9 nm, as shown in Supplementary Fig. 5e,i , the resolution has degraded as compared with the monochromated image, thus the triangle–hexagon structure might appear like a five-membered ring, with the outermost atom appearing brighter than the rest. The sample height was continuously adjusted by a piezo controller to maintain a defocus value of ~1 nm. Holes were created in graphene using a focussed electron beam with BCD of ~1 × 10 8 e s −1 nm −2 with several minutes exposure time. Once a small hole was created, the beam is expanded to a reduced BCD of ~0.1–1 × 10 6 e s −1 nm −2 and images are acquired. Under these ‘imaging’ BCD conditions, the hole expansion rate is slow with a measured change in hole diameter of 1.38 pm s −1 . This ensures that edge configurations remain constant for several seconds and permit sequential image acquisitions that can be averaged to obtain a final image with high signal-to-noise ratio. The diameter of the electron beam for irradiation during image acquisition is typically between 50–100 nm. The TEM images in Figs 1a and 2a were produced by averaging three consecutive frames where the structure had not changed. First, a FFT band-pass filter between 100 to 1 pixels was used to remove the illumination variation, then the three images were aligned and the average generated using Image J. The resultant image was then smoothed to remove further noise. The colour look-up table ‘Fire’ was used to improve visual contrast. Great care was taken to ensure these processes do not introduce artefacts in the final image. Multi-slice image simulations were performed using JEMS software with supercells. The supercell structures were created using Accelrys Discovery Studio Visualizer with atomic coordinates generated from DFT calculations. Supplementary Fig. 7 shows how boxed line profiles are used to measure the distance between neighbouring atoms. The graphene lattice is separated into its three relevant directions, shown by boxes 1, 2 and 3. First, a hexagon (that is, six carbon atoms forming six C–C bonds) is chosen in a region away from the edge and the six C–C bonds are measured by a boxed line profile. This yields two C–C bond lengths per lattice direction and the average of these two values is used as the reference C–C bond length for that specific direction. Next, all the C–C bond lengths are measured across the image and then divided by their directional-specific reference C–C bond length. This removes the effect of residual aberrations because the reference C–C bond experiences the same aberrations as all other C–C bonds in the same direction and by calculating the ratio of the two C–C bond lengths we eliminate this. This process does not work for defects involving Stone–Wales rotations, pentagons or heptagons, where the bond directions are not parallel to one of the three lattice directions and thus there is no suitable reference C–C bond to use. DFT calculations We perform DFT total energy calculations to obtain hydrogen-free and hydrogen-terminated edge structure in graphene. The DFT calculations are performed within the generalized gradient approximation of Perdew–Burke–Ernzerhof functional using Vienna ab initio simulation package (VASP) code [36] , [37] . The basis set contains plane waves up to an energy cutoff of 400 eV. The unit cell is constructed by removing 52 carbon atoms from pristine graphene of 448 carbon atoms to make a hole and edges. In the case of hydrogen-terminated edge structure, 18 hydrogen atoms are attached at the edge of the hole. In constructing the supercell for simulation, we contain a vacuum region of 30 Å in the z direction. The Brillouin zone was sampled using a (2 × 2 × 1) Γ-centred mesh. When structural relaxations are performed, the structure is fully relaxed until the force on each atom is smaller than 0.02 eV/Å. TBMD simulation The TBMD simulations are performed using a modified environment-dependent tight-binding (EDTB) carbon potential, which was modified from the original EDTB carbon potential to study carbon sp 2 bond networks [38] , [39] . This modified EDTB carbon potential has been successfully applied to investigations of various defect structures in graphene [40] , [41] . Details of TBMD simulation methods have been described in previous papers [38] . In TBMD simulations, the self-consistent calculations are performed by including a Hubbard- U term in TB Hamiltonian to describe correctly charge transfers in carbon atoms of dangling bonds and to prevent unrealistic overestimation of charge transfers. The equations of motions of the atoms are solved by the fifth-order predictor–corrector algorithm with a time step of 1.0 fs. All simulations are started at temperature of 2,500 K under the canonical control of temperature. The temperature is gradually increased to 3,200 K under the linear temperature control to accelerate the dynamics so that structural changes at edge can be observed during the simulation time. The velocity scaling method was also used to control the temperature. In the simulation unit cell, we removed 102 carbon atoms from pristine graphene of 364 carbon atoms to make a hole and edges. How to cite this article: He, K. et al. Hydrogen-free graphene edges. Nat. Commun. 5:3040 doi: 10.1038/ncomms4040 (2014).